Prominent electrochromism through vacancy-order melting in a complex oxide Electrochromes are materials that have the ability to reversibly change from one colour state to another with the application of an electric field. Electrochromic colouration efficiency is typically large in organic materials that are not very stable chemically. Here we show that inorganic Bi 0.9 Ca 0.1 FeO 3−0.05 thin films exhibit a prominent electrochromic effect arising from an intrinsic mechanism due to the melting of oxygen-vacancy ordering and the associated redistribution of carriers. We use a combination of optical characterization techniques in conjunction with high-resolution transmission electron microscopy and first-principles theory. The absorption change and colouration efficiency at the band edge (blue-cyan region) are 4.8×10 6 m −1 and 190 cm 2 C −1 , respectively, which are the highest reported values for inorganic electrochromes, even exceeding values of some organic materials. Electric-field-induced phase transitions from a glassy disordered state to an ordered polar state are well known in liquid crystals both with applied DC and AC electric fields [1] , [2] . In the present work, we discover an analogous process in oxide dielectrics, which results in a new electrochromic effect of sufficient strength for commercial devices. Electrochromism has been found in both organic and inorganic materials, each with varying sets of colours. The ability to change material colours with applied electric fields has found several commercial applications in smart windows, goggles, and displays. Most of these electrochromic devices involve doped transition metal oxides, such as WO 3 and chemically substituted derivatives of this material, in which an electrochemical redox reaction leads to the change in colour [3] , [4] , [5] , [6] , [7] , [8] , [9] , [10] , [11] . In recent years, multicomponent transition metal oxides, such as the perovskite manganites, ferroelectric Pb[Zr x Ti (1− x ) ]O 3 and, more recently, the multiferroic BiFeO 3 (BFO) have demonstrated a much broader range of chemical, structural and functional tunability. This arises naturally out of the fact that the two sub-lattices in the perovskite structure can be independently tuned through chemical substitutions, leading to significant changes in functional responses. For example, in the BFO system, ferroelectricity arises primarily from the large polarizability of the 6 s electrons on the Bi site whereas antiferromagnetic order arises from the superexchange interactions among the Fe-ions mediated through the oxygen ions. The optical properties of such systems are typically set by the transition metal 3 d to O 2 p electronic transitions. With this as the background, we are beginning to explore the optical responses of doped perovskites that can be controlled through electric fields. In this paper, we demonstrate a mechanism of intrinsic electrochromic behaviour, in a doped ferroelectric Bi 0.9 Ca 0.1 FeO 3−0.05 (BCFO), caused by changes in carrier density because of the melting of the intrinsic oxygen vacancy order and the resulting oxygen vacancy redistribution. The observed effect is large compared with effects in other transition-metal-oxide electrochromes. Bismuth ferrite has gained interest because a paper published in 2003 showing a large remnant polarization [12] . It has an optical band gap of 2.7 eV (ref. 13 ). The material is multiferroic at room temperature, holds promise for applications in magnetic memory devices, and shows interesting photovoltaic properties [14] . Previously, studies have been done on domain-inversion and electrical modulation of conductance and memristive switching in multiferroic Ca-doped BFO thin films [15] . It was found that the mechanism of this modulation was due to the movement of compensating oxygen vacancies. It was shown that the calcium in BCFO occupies the Bi-lattice position. As Ca 2+ and Bi 3+ differ in valence, the dopant causes the spontaneous formation of oxygen vacancies to maintain balanced valences. With the application of an electrical bias, these oxygen vacancies diffuse towards the negative electrode because of their net positive charge. This migration forms two regions, one that is rich in oxygen vacancies and one that is poor, which essentially forms n-type and p-type conductors, respectively. Hence, in the present work, we modulated the conductance of BCFO films by applying an electric field to redistribute the oxygen vacancies and explore the film's electrochromic properties. Optical and electrochromic characterization Calcium-doped bismuth ferrite thin films of 100 nm thickness were grown epitaxially on strontium titanate (SrTiO 3 ) substrates via pulsed laser deposition with and without strontium ruthenate (SrRuO 3 ) bottom electrodes, as described in previous work [12] , [15] . X-ray diffraction was used to verify the high quality of the epitaxial thin films. In addition, macroscopic optical absorption measurements were performed. A plot of αE 2 versus photon energy E and the linear extrapolation to αE 2 =0 indicates a direct gap at 2.5 eV for Bi 0.9 Ca 0.1 FeO 3−0.05 , as shown in Fig. 1a . This value is slightly lower than that obtained for pure BFO [13] . 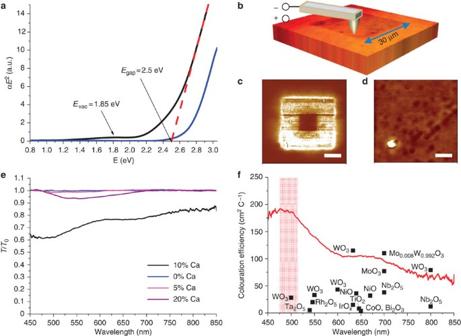Figure 1: Optical and electrochromic characterization. (a) Optical bandgapEg=2.5 eV (red dashed line) of Bi0.9Ca0.1FeO3−0.05evaluated from absorption measurement (black). An additional absorption band originating from oxygen vacancies is visible aroundEvac=1.85 eV. Data for BFO is shown for comparison (blue). (b) Schematic of conductive AFM poling of the sample at −12 V, and optical microscope image (×40) of a 30-μm by 30-μm poled region in a 100-nm thick film. (c) Conductive AFM image of a double box poled with −12 V/+12 V. Scale bar, 1 μm. (d) Topography image of the same area after poling showing no morphology change. Scale bar, 1 μm. (e) Transmission change versus wavelength for different Ca-doping levels (T–transmission inside poled box,T0—transmission outside poled box). (f) Colouration efficiency versus wavelength for Bi0.9Ca0.1FeO3−0.05(red). Maximum CE is 190 cm2C−1at 480 nm (2.55 eV, pink area). Values for known inorganic electrochromic materials are added for comparison; absolute values are shown (data points adapted from ref.5). Figure 1: Optical and electrochromic characterization. ( a ) Optical bandgap E g =2.5 eV (red dashed line) of Bi 0.9 Ca 0.1 FeO 3−0.05 evaluated from absorption measurement (black). An additional absorption band originating from oxygen vacancies is visible around E vac =1.85 eV. Data for BFO is shown for comparison (blue). ( b ) Schematic of conductive AFM poling of the sample at −12 V, and optical microscope image (×40) of a 30-μm by 30-μm poled region in a 100-nm thick film. ( c ) Conductive AFM image of a double box poled with −12 V/+12 V. Scale bar, 1 μm. ( d ) Topography image of the same area after poling showing no morphology change. Scale bar, 1 μm. ( e ) Transmission change versus wavelength for different Ca-doping levels ( T –transmission inside poled box, T 0 —transmission outside poled box). ( f ) Colouration efficiency versus wavelength for Bi 0.9 Ca 0.1 FeO 3−0.05 (red). Maximum CE is 190 cm 2 C −1 at 480 nm (2.55 eV, pink area). Values for known inorganic electrochromic materials are added for comparison; absolute values are shown (data points adapted from ref. 5 ). Full size image For the investigation of electrochromism, we use a home-built optical set-up incorporating a white-light source (tungsten lamp) and a visible to near-infrared spectrometer (Ocean-Optics USB400), for local optical absorption spectroscopy. Objective lenses were utilized to obtain a beam spot size of less than 20 μm when focused onto the sample. Micrometre-sized regions of the Ca-doped BFO thin films were poled using a Veeco conductive atomic force microscope, as described in previous work and seen in Fig. 1b (ref. 15 ). Several 30 μm by 30 μm boxes were poled with a bias of −12 V and tip velocity of 3 μm s −1 while the current of the region was monitored. The film surface was also monitored to ensure that there was no damage. Poling was stopped when the current reached about 1 μA. A CCD camera attached to the aforementioned optical set-up was sufficient in finding the poled boxes to align for absorption spectroscopy. The spectra were analysed at various spots outside the written boxes and compared with that of inside the box. Figure 1b shows the visible change of the sample surface as seen through a microscope after conductive atomic force microscopy (c-AFM) poling. Great care was taken to avoid the dielectric breakdown regime during electrical poling. In the case of every measured dataset, the increased electrical conductivity and the surface morphology of the poled area was checked and found pristine after poling. An example is shown in Fig. 1c,d . This method produced rather consistent results, and visible spectra data was acquired. Furthermore, annealing the samples at 150 °C for 4 h caused the boxes to visibly disappear completely. This is due to an increase in diffusivity of the oxygen vacancies allowing them to spread throughout the material back to their equilibrium, thereby lowering the effective free carrier density. Figure 1e shows the transmission change after poling of the material as a function of wavelength. The reference spectrum T 0 is taken to be the transmittance of the uncoloured region of the BCFO film outside of the electrically poled box shown in Fig. 1b . The minimum transmission for 10% Ca doping occurs at 2.55 eV (485 nm), which is approximately the band gap, E g , of BCFO. The change in visible transmittance spectra at this wavelength is 40%. Additionally, there is a small minimum at about 670 nm (1.85 eV), which is associated with oxygen vacancies in the sample. From the transmission change, Δ T=T/T 0 , the absorption coefficient and colouration efficiency (CE) are calculated. The absorption coefficient is evaluated from: where t is the film thickness. At 480-nm wavelength, Δα is calculated to be 4.8×10 6 m −1 . The CE is evaluated from: where Q is the volumetric charge density. To calculate Q , we must take some assumptions compared with a typical electrochromic device because charge is not injected into the system, but rather formed intrinsically through charge separation. We neglect all diffusion gradients and assume that there are two half spaces to the film: an n-type and a p-type region. We also assume that all oxygen vacancies have fully diffused, and the number of oxygen vacancies per unit volume, n Vo , after doping and before c-AFM, is constant, each contributing two electron carriers when diffused. As we know only the p-type region contributes to the colouration change [15] , we make a conservative estimate that the absorption changes in the p-type region equals to the measured effective absorption change. For the p-type region, each missing oxygen vacancy produces two holes making the carrier density produced in the volume equal to 2 n Vo . These assumptions allow us to find the theoretical lower bound on CE for the measured α at a given wavelength. In our previous work, we found that the initial oxygen vacancy density n Vo for Bi 0.9 Ca 0.1 FeO 3−0.05 is 8×10 20 cm −3 (ref. 15 ) implying that the volumetric charge density, Q , is 2.5632×10 8 m −3 C. At 480-nm wavelength, CE is calculated to be 190 cm 2 /C ( Fig. 1f ). This value is higher than CEs found in most transition-metal-oxide electrochromes; it even surpasses CE values reported for organic electrochromes, such as indigo blue, which usually show higher CE values than inorganic materials, but are less chemically stable [5] . For a comparison of colouration efficiencies of oxide electrochromes, see Fig. 1f . Transmission electron microscopy studies The absorption change for 20% Ca is smaller than that for 10% Ca, as seen in Fig. 1e . If only the absolute amount of oxygen vacancies present determined the effect, one would intuitively expect the opposite to be the case. Clearly, there must be some microscopic difference in both types of samples that leads to the observed behaviour. To gain more insight, we performed high-resolution transmission electron microscopy (TEM) studies of both 10 and 20% Ca-doped BFO samples in the as-grown and poled states. The results are seen in Fig. 2 . 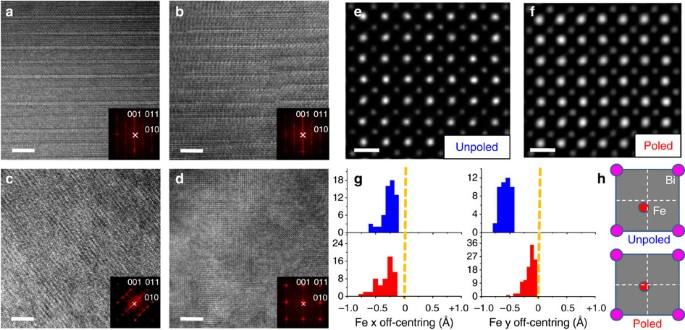Figure 2: TEM characterization of the oxygen-vacancy ordering in Ca-doped BFO. (a) Ca 20% as-grown, (b) Ca 20% poled, (c) Ca 10% as-grown, (d) Ca 10% poled; scale bars, 5 nm, insets show local diffraction patterns. (e,f) High resolution TEM showing ion positions for poled and unpoled state for Ca 10% (scale bars, 0.4 nm). (g) Histogram analysis of Fe ion position. Dashed yellow lines indicate the centre of the unit cell. (h) Schematic of Fe-ion displacement using data of (g). Figure 2a shows the as-grown state of a sample containing 20% Ca. The oxygen-vacancy order parallel to the sample surface with a period of eight unit cells is seen. An image of the c-AFM-poled state after application of −12 V can be seen in Fig. 2b . The application of an electric field does not yield changes in the oxygen-vacancy ordering. Figure 2: TEM characterization of the oxygen-vacancy ordering in Ca-doped BFO. ( a ) Ca 20% as-grown, ( b ) Ca 20% poled, ( c ) Ca 10% as-grown, ( d ) Ca 10% poled; scale bars, 5 nm, insets show local diffraction patterns. ( e , f ) High resolution TEM showing ion positions for poled and unpoled state for Ca 10% (scale bars, 0.4 nm). ( g ) Histogram analysis of Fe ion position. Dashed yellow lines indicate the centre of the unit cell. ( h ) Schematic of Fe-ion displacement using data of ( g ). Full size image The results for the same type of measurements for a sample containing 10% Ca are shown in Fig. 2c,d . The as-grown state shows an oxygen-vacancy ordering with a period of 2–3 unit cells under an angle of 45° to the sample surface. After the application of a bias of −12 V in the c-AFM poling, the oxygen-vacancy ordering is completely melted. In this area, the overall vacancy concentration is lowered after poling, whereby the area becomes p-type [15] . A close inspection of the individual ion positions for the poled and unpoled state, by high-resolution TEM, is presented in Fig. 2e,f . From these images, Fe-ion position coordinates were extracted as shown in Fig. 2g . Histogram plots show that the average Fe off-centring is reduced for the poled state as compared with the unpoled state. A schematic representation can be seen in Fig. 2h . In addition, at high temperature, the measured band gap of BFO decreases as the deviation from the cubic structure decreases [16] , [17] . Both studies indicate that the optical properties of undoped BFO are sensitive to the polar order parameter and the structural symmetry. In our case, the strong electrochromic colouration in the electrically poled state is accompanied by a relative shift of the Fe ion with respect to the unit cell centre also indicating a change of the polar order parameter. First principles calculations To understand the effects of calcium doping and oxygen vacancies on the optical properties of BFO, for both the compensated and p-type case, we have also performed first-principles density-functional theory [18] , [19] (DFT) calculations, using approaches previously used for BFO [20] , [21] , [22] , [23] , [24] , [25] (Methods). After the structural and electronic ground states have been determined, the frequency-dependent real part ε 1 and imaginary part ε 2 of the dielectric function are calculated [26] . The usual expression for the optical absorption coefficient α( ω ) is, where ω is the energy of the absorbed photon, n is the refractive index, and c 0 is the speed of light in vacuum. The optical absorption coefficient α( ω ) can also be expressed in terms of the real and imaginary parts of the dielectric function, The calculated electronic density-of-states and optical absorption coefficients of both the uncompensated and the compensated Ca-doped BFO are shown in Fig. 3a,b . It is well known that density functional theory calculations underestimate the band gap for most materials, and incorporation of onsite Coulomb interaction with Hubbard U parameter improves the band gap value. It has also been shown that oxygen vacancies have a role in the optical properties of BFO [25] . With the specific choice of onsite Coulomb interaction parameters ( U =4 eV, J =1 eV), the optical band gap is calculated to be 1.95 eV for undoped BFO. Assuming 1/8 of Ca doping and complete compensation of holes by oxygen vacancies (Ca 1/8 Bi 7/8 FeO 3−1/16 in Fig. 3 ), the optical band gap is reduced by 0.1 eV from the undoped material. This result is consistent with our experimental observations, which show that Ca doping reduces the band gap of BFO from 2.7 (ref. 13 ) to 2.5 eV ( Fig. 1a ). Because of the complete charge compensation, the Fermi level lies in the band gap. Ca-doped BFO without charge compensation from oxygen vacancies shows a much sharper rise in the density-of-states of the conduction band, which results in an enhanced optical absorption near the band edge (Ca 1/8 Bi 7/8 FeO 3 in Fig. 3a ). The difference between the compensated and the uncompensated Ca-doped BFO, in the density-of-states of the conduction bands, becomes apparent by looking at the electron density of the lowest conduction states, as shown in Fig. 3c,d . The lowest conduction states in uncompensated Ca-doped BFO are mostly extended Fe 3d states, similar to undoped BFO. In contrast, the lowest conduction states in compensated Ca-doped BFO localize at Fe sites near the compensating oxygen vacancies. 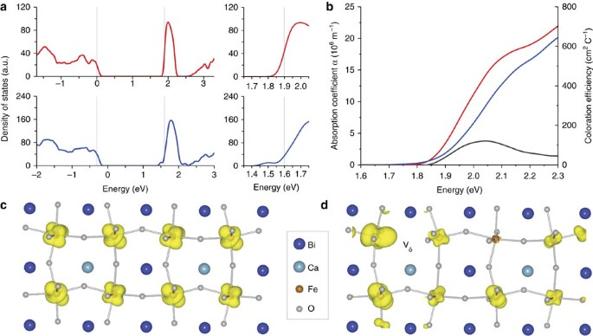Figure 3: First-principles calculations. (a) Calculated electronic density-of-states near the bandgap (blue lines) for BFO with calcium doping Bi7/8Ca1/8FeO3(red) and BFO with calcium doping and oxygen vacancy compensation Ca1/8Bi7/8FeO3−1/16(blue). (b) Optical absorption coefficientsαas a function of photon energy. The calculations are performed using GGA+Umethod withU=4 eV andJ=1 eV for BFO with calcium doping Bi7/8Ca1/8FeO3(red) and BFO with calcium doping and oxygen-vacancy compensation Ca1/8Bi7/8FeO3−1/16(blue). Calculated CE is also shown (grey). (c) Isosurface electron density of the lowest lying conduction band states in coloured Bi7/8Ca1/8FeO3, and (d) in oxygen-vacancy compensated Ca1/8Bi7/8FeO3−1/16(Vödenotes position of oxygen vacancy (Kröger–Vink notation)). Figure 3: First-principles calculations. ( a ) Calculated electronic density-of-states near the bandgap (blue lines) for BFO with calcium doping Bi 7/8 Ca 1/8 FeO 3 (red) and BFO with calcium doping and oxygen vacancy compensation Ca 1/8 Bi 7/8 FeO 3−1/16 (blue). ( b ) Optical absorption coefficients α as a function of photon energy. The calculations are performed using GGA+ U method with U =4 eV and J =1 eV for BFO with calcium doping Bi 7/8 Ca 1/8 FeO 3 (red) and BFO with calcium doping and oxygen-vacancy compensation Ca 1/8 Bi 7/8 FeO 3−1/16 (blue). Calculated CE is also shown (grey). ( c ) Isosurface electron density of the lowest lying conduction band states in coloured Bi 7/8 Ca 1/8 FeO 3 , and ( d ) in oxygen-vacancy compensated Ca 1/8 Bi 7/8 FeO 3−1/16 ( V ö denotes position of oxygen vacancy (Kröger–Vink notation)). Full size image The defect-like localized states in compensated BCFO correspond to the small shoulder at the conduction band edge in the electronic density-of-states, resulting in the reduced density-of-states of the extended conduction band states just above it ( Fig. 3a ) and the lower optical absorption coefficient near the band edge. At 1.95 eV, the difference in calculated absorption coefficient is 3.4×10 6 m −1 , which is in very good agreement with the measured change of 4.8×10 6 m −1 at 480 nm. The theoretical calculations and the TEM characterization point to the following mechanism of colossal electrochromism in 10% Ca-doped BFO. In the as-grown sample, oxygen vacancies compensate the Ca dopants and form ordered structures. On application of an electric field, the vacancy ordering is melted, and vacancy-rich (n-type) and poor (p-type) regions are formed owing to the resulting redistribution of vacancies. The large colouration originates from the increased optical absorption at the band edge of the p-type region. In contrast, oxygen-vacancy ordering in 20% Ca-doped BFO remains almost unchanged under an electric field, which is consistent with the small change in absorption. DFT calculations were carried out with supercells containing uniformly distributed Ca dopants and oxygen vacancies. The effects of extended oxygen vacancies such as vacancy clusters or planes of ordered vacancies, observed in other transition metal oxides, have not been explored theoretically in the current study because of the high computational demand. However, a recent study has shown that oxygen vacancy clustering in SrTiO 3 induces localized states at 0.6 eV below the conduction band minimum [27] , whereas the single vacancy states are much closer to the conduction band minimum. The observed weak absorption peak at 1.85 eV in our measurements could therefore also originate from clustering of oxygen vacancies. Our experimental and theoretical studies have revealed a new kind of electrochromic phenomenon. In comparison with earlier work, electrochromic work on WO 3 usually involves samples with nanocrystals embedded in a glassy matrix, and coupled cation and electron transport occurs over large distances and is confined to the non-crystalline matrix [28] ; and in crystalline SrTiO 3 (ref. 29 ), ionic transport requires exotic valence states of Ti (and/or Sr). Of particular interest, from the electrochromics point of view, is that the present system involves local oxygen ordering within a crystalline state, which is unlikely to require exotic valences while still achieving large intrinsic electrochromic effects. The ability to reversibly achieve a large change in visible transmittance in the blue-cyan region (2.55 eV) is so far unmatched in transition metal oxides. Our observations support the notion that such behaviour accompanied by a structural transition as seen in a change of Fe-ion displacement is a generic feature akin to chemically driven phase changes that are now well established in complex oxide systems such as manganites, cuprates, and relaxor materials [30] . Furthermore, the observation of strong absorption change and colouration, that is achieved solely by redistribution of oxygen vacancies within the material itself, by melting the vacancy-ordered state, should motivate a search for similar control in other related complex oxide systems, thus making this intrinsic effect potentially attractive for electrochromic device applications. Materials X-ray characterization High-resolution X-ray reciprocal space mapping studies were completed on a Bi 0.9 Ca 0.1 FeO 3−0.05 (BCFO) film (~300 nm in thickness) grown on (001) SrTiO 3 substrates using a Panalytical X'Pert MRD Pro 4-circle diffractometer ( Fig. 4 ). We measured the (203) peak to investigate the in-plane lattice parameter as well as the out-of-plane lattice parameter. The (203) diffraction peak of the film is located near the dashed line indicating the film has been grown coherently and, thus, the in-plane lattice parameter of the film is nearly identical to that of the substrate. However, the shape of the peak is somewhat diffused along the transverse scan direction as a result of partial strain relaxation which is natural in such a thick (~300 nm) film. Normal BFO films show the split of the (203) peak arising from monoclinic distortion of the unit-cell; however, this BCFO film does not show any peak split indicating that the unit cell is ideally tetragonal. From the (203) peak position, we can calculate the lattice parameters of the unit-cell to be a =3.906 Å and c =3.941 Å. The structural analysis confirms that the BCFO film has been grown epitaxially on (001) SrTiO 3 substrate, and the stabilized phase can be described by a tetragonal unit cell. 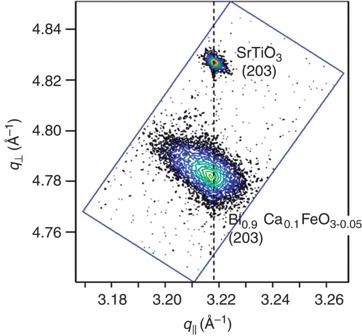Figure 4: X-ray diffraction structural characterization. X-ray reciprocal space map of an epitaxially grown Bi0.9Ca0.1FeO3−0.05film. Figure 4: X-ray diffraction structural characterization. X-ray reciprocal space map of an epitaxially grown Bi 0.9 Ca 0.1 FeO 3−0.05 film. Full size image Transmission electron microscopy High-angle annular dark-field scanning transmission electron microscopy was carried out using the aberration-corrected TEAM 0.5 microscope (a modified FEI Titan 80–300 quipped with a Schottky-type high-brightness field-emission electron source and an improved hexapole-type spherical aberration (CS) corrector) located at the National Center for Electron Microscopy (NCEM). The TEAM 0.5 microscope was operated at 300 kV. The probe semi-convergence angle was set to 16.5 mrad, which yields a calculated probe size of 0.63 Å. Although a smaller probe size is in principle feasible on the expenses of a reduced depth of field, the chosen setting allows for a sufficiently large depth of field, which enhances the contrast of the atomic columns. The annular semidetection range of the high-angle annular dark-field detector was about 45–290 mrad. Atomic force microscopy Local electrical poling under ambient conditions was achieved using an AFM-based set-up. Measurements were carried out on a Digital Instruments Nanoscope-IV Multimode AFM equipped with a conductive AFM application module. The investigations were carried out with commercially available nitrogen-doped diamond-coated Si tips (NT-MDT). Typical scan rates were 3 μm s −1 . First-principles calculations We perform first-principles density-functional theory calculations using the projector-augmented-wave method as implemented in the Vienna ab-initio software package code. Density-functional theory with generalized-gradient approximation plus onsite Coulomb interaction (GGA+ U ) is used with parameters U =4 eV and J =1 eV, which is within the range of values used in the literature. We use a 500-eV plane-wave cutoff energy for both structural optimization and dielectric function calculations. The lattice of bulk BFO has rhombohedral symmetry with G-type AFM order. Supercells containing 2×2×2 or 2×2×4 pseudo-cubic perovskite units are used for simulating Ca-doping and oxygen vacancies. The ionic positions are relaxed so that the force on every ion is less than 10 meV Å −1 . The frequency dependent dielectric function is calculated after the structural and electronic ground states have been determined. How to cite this article: Seidel, J. et al . Prominent electrochromism through vacancy-order melting in a complex oxide. Nat. Commun. 3:799 doi: 10.1038/ncomms1799 (2012).